Structure units oriented approach towards collective synthesis of sarpagine-ajmaline-koumine type alkaloids 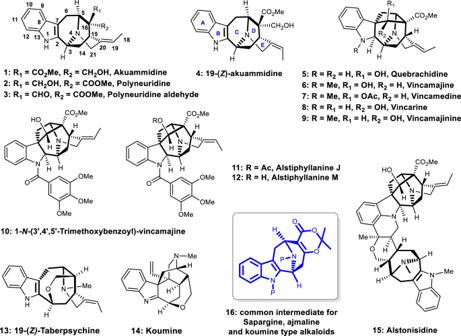Fig. 1: Some representative sarpagine-ajmaline-koumine type alkaloids. In this work, alkaloids1–9,11,13, and14are synthesized. Sarpagine-Ajmaline-Koumine type monoterpenoid indole alkaloids represent a fascinating class of natural products with polycyclic and cage-like structures, interesting biological activities, and related biosynthetic origins. Herein we report a unified approach towards the asymmetric synthesis of these three types of alkaloids, leading to a collective synthesis of 14 natural alkaloids. Among them, akuammidine, 19- Z -akuammidine, vincamedine, vincarine, quebrachidine, vincamajine, alstiphylianine J, and dihydrokoumine are accomplished for the first time. Features of our synthesis are a new Mannich-type cyclization to construct the key indole-fused azabicyclo[3.3.1]nonane common intermediate, a SmI 2 mediated coupling to fuse the aza-bridged E-ring, stereoselective olefinations to install either the 19- E or 19- Z terminal alkenes presented in the natural alkaloids, and an efficient iodo-induced cyclization to establish the two vicinal all-carbon quaternary centers in the Koumine-type alkaloids. The sarpagine alkaloids feature a polycyclic ring system with an azabicyclo[3.3.1]-nonane core. These alkaloids serve as the biogenetic precursors for the more complex ajmaline and koumine type indole alkaloids [1] , [2] , [3] . The sarpagine-ajmaline-koumine type alkaloids are among the most important group of monoterpenoid indole alkaloids [4] , [5] , [6] . Those biogenetically related alkaloids have been isolated mainly from the medicinal plant family Apocynaceae and Loganiaceae, especially from the genera Alstonia , Rauwolfia, and Gelsemium in low natural abundance [7] , [8] , [9] , [10] . A number of these alkaloids possess important biological activities, including anti-leishmanial [11] , anti-malaria parasites [12] , anti-inflammatory [13] , antihypertensive [14] , anticancer [15] , and accelerating the sciatic nerve regeneration activities [16] . The typical molecules are indicated in Fig. 1 . Because of their characteristic indole-fused azabicyclo[3.3.1]-nonane structures and prominent biological activities, sarpagine-ajmaline-koumine related alkaloids have attracted attention from the organic synthetic community for decades [17] , [18] , [19] , [20] , [21] , [22] , [23] , [24] , [25] . Synthetic efforts have resulted in a number of elegant strategies and culminated with the synthesis of a series of sarpagine˗ajmaline-koumine type alkaloids. Formation of the indole fused azabicyclo[3.3.1]nonane structures could be roughly classified to five categories: the Pictet-Spengler cyclization (forming the C2-C3 bond) approaches, the intramolecular condensation/addition methodologies (constructing the C15-C16 bond), the transition metal-mediated cyclizations, the cycloaddition/annulation strategies, and the Friedel-Crafts acylation approach (forming the C6-C7 bond). The first category includes Tamelen’s [26] , Masamune’s [27] , Craig’s [28] , Sudhakar’s [29] Pictet-Spengler cyclization procedures, and most recently, Qi’s aza-Achmatowicz rearrangement of indole-tethered furan followed by Pictet-Spengler cyclization [30] . The second category constitutes Cook’s approach based on Dieckman condensation of carboline derivatives [31] , [32] , [33] , [34] , [35] , [36] , [37] , [38] , [39] , [40] , [41] , [42] , and Bailey’s intramolecular Michael addition procedures [43] , [44] . The third category comprises Martin’s approach via Pauson-Khand reaction [45] , olefin metathesis [46] , Kuethe’s intramolecular Heck cyclization approach [47] , and most recently, Zhang’s Copper-catalyzed oxidative cyclization [48] , [49] . The fourth category includes Ohba’s intramolecular oxazole–olefin Diels–Alder cycloaddition [50] , and Gaich’s [5 + 2] cycloaddition followed by ring enlargement and Fischer indole annulation [51] , [52] , [53] . The last category is Kwon’s intramolecular Friedel-Crafts acylation approach [54] . Numerous sarpagine˗ajmaline-koumine type alkaloids have been synthesized based on above-mentioned strategies, however, quebrachidine, vincamedine, and its analogues are not yet conquered to our knowledge by total synthesis [17] , [18] , [19] , [20] , [21] , [22] , [23] , [24] , [25] . The natural alkaloid quebrachidine ( 5 ) and its N -methyl congener vincamajine ( 6 ) and vincamedine ( 7 ) are among the most highly functionalized and synthetically challenging ajmaline type alkaloids. Quebrachidine is the biogenetic precursor of bisindole alkaloid alstonisidine ( 15 ) and has been isolated for more than 50 years [55] , while vincamedine and alstiphyllanines (Fig. 1 , 11 and 12 ) possess potent vasorelaxant activity [56] . It is also noteworthy that alstiphyllanines are 19- Z -derivatives of quebrachidine. Fig. 1: Some representative sarpagine-ajmaline-koumine type alkaloids. In this work, alkaloids 1 – 9 , 11 , 13 , and 14 are synthesized. Full size image In this work, we report a structure-unit-oriented strategy towards the synthesis of 14 natural monoterpenoid indole alkaloids. Although numerous synthetic methods have been developed for sarpagine-ajmaline alkaloids as well as structurally related analogues, flexible and unified synthetic routes that lead to collective synthesis of these types of alkaloids, especially towards both 19- E and 19- Z isomers, are rarely documented [17] , [18] , [19] , [20] , [21] , [22] , [23] , [24] , [25] . Retrosynthetic analysis As part of our ongoing program in seeking flexible and divergent synthetic strategies toward bioactive natural products and its analogues [57] , [58] , [59] , [60] , [61] , we recently disclosed a Lewis acid-mediated intramolecular Prins reaction of dioxinones to construct medium-sized carbocycles bearing oxa-bridged bicyclic structural units [62] . We envisioned that the Mannich-type-cyclization version of our previous protocol might lead to the highly functional 9-azabicyclo[3.3.1]nonane ring system ( 16 , Fig. 2 ), an ideal intermediate with properly located functional groups and necessary carbons for the synthesis of akuammidine-related alkaloids shown in Fig. 1 . Fig. 2: Retrosynthetic analysis based on amide-mediated Mannich-type cyclizations. The collective synthesis of sarpagine-ajmaline-koumine type alkaloids are based on common intermediate 16 . Full size image Our retrosynthetic analysis is outlined in Fig. 2 . One of the key transformations in the synthetic plan is cascade cyclizations (Fig. 2 , transformation of 19 → 16 ) to form the aza-bridged eight-membered ring system from indole fused chain compound ( 19 ). Although we have succeeded previously the synthesis of oxa-bridged medium-sized ring systems [62] , and aza-Prins cyclization have been used elegantly in the synthesis of six-membered carbocyclic rings [63] , [64] , the proposed tandem cyclizations to obtain aza-bridged bicyclo[3.3.1]nonane common structure units ( 16 ) are challenging. We postulated that an amine or amide participated intramolecular Mannich-type reaction of dioxinones under Lewis acid conditions would provide access to the required common intermediate ( 16 , Fig. 2 ). Based on the well-located functional groups, with proper manipulations, we would be able to synthesize the natural alkaloids shown in Fig. 1 . Preparation of the common azabicyclo[3.3.1]-nonane core We commenced our synthetic studies with the preparation of tert -butanesulfinamide 19a (Fig. 3 ). The desired sulfinamide 19a was obtained after two steps in 63% yield from known aldehyde 17a , obtained two steps from commercially available tryptophol [65] . Our initial plans were oxidation of sulfinamide 19b (after removal of PMB with DDQ) or amine 19c (after removal of PMB with DDQ and the tert- butanesulfinyl group with iodine [61] ) to its corresponding aldehydes and subjected it to the proposed Mannich-type reactions. Unfortunately, both substrates ( 19b and 19c ) failed to yield reasonable amounts of aldehydes under a number of oxidation conditions. To circumvent this problem, the amine was converted to amide 19d with Boc-anhydride (71% overall yields in three steps from 19a ). Oxidation of alcohol 19d with IBX [66] provided an unstable aldehyde ( 19e ), which was used immediately in the cyclization under Lewis acid conditions. To our delight, the cascade sequence proceeded precisely and produced the desired 16a as a single diastereoisomer in 57% yield (gram-scale) over two consecutive steps. The correct stereochemistry of the pentacyclic core was confirmed by single crystal X-ray analysis. Fig. 3: Gram-scale synthesis of common intermediate 16a. The key transformations to access the common intermediate 16a include a vinylogous Mannich reaction of lithium dienolate 18 , and a Lewis acid mediated Mannich type cyclization of 19e . Ac acetyl, Boc t -butoxycarbonyl, DCM dichloromethane, DDQ 2,3-dichloro-5,6-dicyano-1,4-benzoquinone, IBX o -iodoxybenzoic acid, LiHMDS lithium bis(trimethylsilyl)amide, PMB p -methoxybenzyl, THF tetrahydrofuran. Full size image With the common intermediate 16a in hand, we next explored the synthesis of sarpagine-ajmaline alkaloids indicated in Fig. 1 , aiming to synthesize both 19- E and 19- Z natural isomers. Treatment of 16a with sodium methoxide afforded methyl ester 20a in 94% yield. Deoxygenation of enol 20a via formation of triflate with Comins reagent followed by palladium-catalyzed hydrogenolysis [67] , [68] provided 20b in excellent yield. Next, the Boc protecting group was removed with trifluoroacetic acid in dichloromethane and the resultant was treated with ( Z )-1-bromo-2-iodobute-2-ene to afford intermediate 20c . Our initial plan to fuse the C 15 -C 20 carbon-carbon bond of akuammidine-related alkaloids was to follow the well-established procedure via reductive Heck-type reactions [69] , [70] , [71] , [72] , [73] , [74] , [75] , [76] . To our dismay, no desired product was obtained under various palladium and nickel mediated conditions, with dehalogenation product being isolated in most cases (see Supplementary Information for details). Treatment of iodide 20c with tri- n -butyltin hydride [77] was also fruitless, with a complex mixture being obtained. Difficulty in assembling the bridged E-ring prompted us to explore alternative methods. It was of our interests to use Skrydstrup’s chemistry [78] , [79] , [80] , [81] , [82] , [83] , [84] , namely SmI 2 mediated acyl radical reaction. As indicated in Fig. 4 , Skrydstrup coupling would lead to a tempting product, namely intermediate 23 , which bears a tunable carbonyl moiety for further manipulation towards desired 19- E and 19- Z olefins. The intermediate 20b was then transformed to its corresponding N -acyl-oxazolidinone derivative 22 (2 steps, 76%). The well-established Skrydstrup’s conditions (SmI 2 /H 2 O/THF) unfortunately failed to promote the desire cyclization, however, after examining several other conditions, we finally established a reproducible procedure for constructing the bridged E-ring (Fig. 4 ). SmI 2 mediated SET reaction gave the coupling product in 76% yield with excellent diastereoselectivity (single C 16 isomers). We deduced that the chelation of samarium diiodide with the carbonyl groups as proposed by Skrydstrup [79] (Fig. 4 ) secured the desired cyclization. The NOESY correlations of H-16 to both H-14 and H-15 for compound 23 indicated a β-orientation of the H-16 (Fig. 4 , see Supplementary Information for spectra). Thus, the pentacyclic skeletons for akuammidine-related alkaloids had been successfully assembled and ready for late-stage manipulation. Fig. 4: Synthesis of the common sarpagine type skeletons. After construction of the bridged E-ring via SmI 2 mediated SET reaction, the double bonds were assembled by Wittig reaction ( E -selectivity) and Julia olefination ( Z -selectivity). DIPEA diisopropylethylamine, DMF N , N -dimethylformamide, HMPA hexamethylphosphoramide, Me methyl, Ph phenyl, TEA triethylamine, Tf trifluoromethanesulfonyl, TFA trifluoroacetic acid, Et ethyl, NaHMDS sodium bis(trimethylsilyl)amide. Full size image We next focused on the selective synthesis of E and Z alkenes with ketone 23 . Treatment of ketone 23 with Wittig reagent [85] , [86] , [87] in THF in the presence of NaHMDS provided olefins 24 (isolated as the major isomer, 83% yield) and 25 (15% yield) in a 98% combined yield. Treatment of ketone 23 with Julia reagent [88] in THF altered the ratio and provided olefin 25 as the major isomer in 80% yield together with 24 (19% yield). Suitable crystal was obtained from compound 25 , and the 19- Z stereochemistry was established by X-ray crystallography (Fig. 4 ). This new approach enabled access to either 19- E (Wittig-olefination, trans -selective) or 19- Z (Julia-olefination, cis -selective) isomers selectively. Total synthesis of natural sarpagine-type and ajmaline-type alkaloids With the advanced intermediates ( 24 and 25 ) in hand, we next began the journey towards akuammidine-related alkaloids. Treatment of 24 with LDA followed by formaldehyde (Fig. 5 ), we obtained desired C16 stereoisomer 26 (55% yield) together with byproduct 27 (17% yield). Using compound 25 , similar operation provided intermediates 28 (42%) and 29 (30%). It is worthwhile to note that the undesired C-16 isomers could be recycled, a retro-Aldol reaction in the presence of sodium hydride converted 27 and 29 back to its corresponding starting materials ( 24 : 86% yield, and 25 : 83% yield, Fig. 5 ). Deprotections of PMB in intermediates 26 and 28 under acidic conditions furnished the first total synthesis of natural akuammidine ( 1 , confirmed by X-ray analysis) and 19- Z -akuammidine ( 4 ). The NMR spectra as well as physical data of our synthetic sample were consistent with those reported in the literature [89] , [90] . Fig. 5: Synthesis of akuammidine (1) and 19- Z -akuammidine (4). Aldol condensation with formaldehyde. LDA lithium diisopropylamide. Full size image Having secured the total synthesis of akuammidines, we next turned our attention to the synthesis of more challenging ajmaline-type alkaloids. To increase the ratio of intermediate 27 , a number of additives were used including BF 3 ∙ Et 2 O, TMSCl (trimethylsilyl chloride), TMEDA ( N , N , N ′, N ′-tetramethylethylenediamine), and HMPA. The addition of HMPA could slightly increase the ratio of compound 27 (30% yield) while undesired C-16 isomer 26 was converted back to starting material ( 24 ) through retro-aldol reaction in 84% yield (Fig. 6 ). Treatment of 27 with TFA in the presence of PhSH yielded natural polyneuridine ( 2 ) in 90% yield [91] , [92] . Corey-Kim oxidation of 2 provided the biosynthetic precursor polyneuridine aldehyde ( 3 ) [3] , [4] , [21] . Upon exposure to acidic conditions (Ac 2 O and TfOH, modification of Cook’s conditions [35] ), an inseparable mixture of C17 stereoisomers ( 30a and 30b , 63% yields in two steps, dr = 1.1:1 based on 1 H-NMR) was obtained. Reduction of the mixture with sodium cyanoborohydride gave amines 31a and 31b (inseparable mixture) in 87% combined yield (Fig. 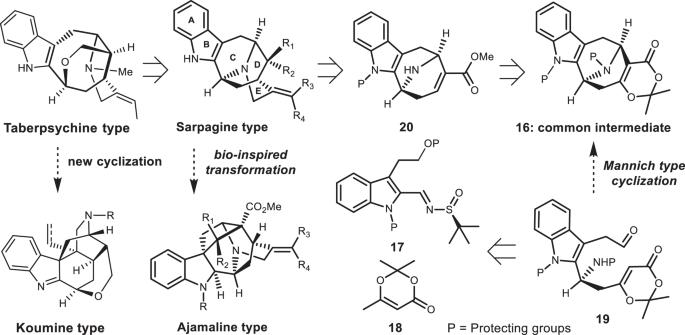Fig. 2: Retrosynthetic analysis based on amide-mediated Mannich-type cyclizations. The collective synthesis of sarpagine-ajmaline-koumine type alkaloids are based on common intermediate16. 6 ). We envisioned that the inseparable C17-acetate isomers might react differently under hydrolysis conditions due to its different steric hindrances. Thus, the mixture of 31a and 31b were treated with K 2 CO 3 in methanol. This process provided unchanged acetate 31a in 50% yield together with natural vincarine ( 8 , 47% yield, from hydrolysis of 31b , the first total synthesis), the diastereoisomer of quebrachidine [6] , [36] , [93] . Reductive amination of 31a with formaldehyde furnished the first total synthesis of vincamedine ( 7 ) [94] . Hydrolysis of 7 afforded vincamajine ( 6 ) [94] in 93% yield. Further hydrolysis of 31a provided the first total synthesis of natural alkaloid quebrachidine ( 5 ) [55] , [95] . The structure of synthetic quebrachidine was confirmed by X-ray crystallography. Fig. 6: Synthesis of ajmaline type alkaloids. Quebrachidine, vincarine, vincamedine, and vincamajine were synthesized for the first time. NCS N -chlorosuccinimide. Full size image Treatment of vincarine ( 8 ) with sodium cyanoborohydride in the presence of formaldehyde gave vincamajinine ( 9 ) [36] . The NMR spectra and physical data of our synthetic samples were in complete agreement with the reported data. It is noteworthy that vincarine has been documented in literature for more than 50 years, no complete reported NMR data are available in the literature [6] , [36] . Next, we concentrated on the total synthesis of alstiphyllanines (with a 19- Z -olefin moiety), a number of bioactive ajmaline-type alkaloids differs from each other only in amide substituents [56] . Aldol reaction of compound 25 (from Julia-olefination in Fig. 4 ) in the presence of HMPA afforded desired isomer 29 in 37% yield (Fig. 7 ). Treatment of 29 with TFA in the presence of PhSH afforded amine 32 in 86% yield. Oxidation of 32 under Corey-Kim conditions gave aldehyde 33 , which was directly subjected to acidic conditions to yield cyclization products 34a and 34b (60% yield over two steps, ∼ 1:1.45 ratio) as an inseparable mixture of C17 diastereoisomers. Selective reduction of the imine moiety presented in 34a and 34b with sodium cyanoborohydride afforded amines 35a and 35b (inseparable mixture of C17 diastereoisomers) in 90% combined yield. Hydrolysis of the mixture of 35a and 35b under our standard conditions provided separable alcohol 36 (59%) and acetate 35a (37%). The alcohol 36 could be recycled by oxidation with MnO 2 in dichloromethane [96] . Finally, treatment of 35a with eudesmoyl chloride in pyridine furnished the first total synthesis of alstiphyllanine J ( 11 ). The NMR spectra of our synthetic sample agree well with the reported data [56] . Fig. 7: Synthesis of alstiphyllanine J. Alstiphyllanine J has a 19- Z -olefin moiety. DMAP N , N -4-dimethylaminopyridine. Full size image Total synthesis of natural koumine-type alkaloids Finally, to further demonstrate the flexibility of our strategy, we decided to synthesize the challenging koumine-type alkaloids, a cage-like alkaloid family with two vicinal all-carbon quaternary centers [5] . There are two key issues in the synthesis of koumine-type alkaloids from common intermediate 25 , namely the epimerization of the C-16 stereochemistry and a cyclization to form the two vicinal all-carbon quaternary centers. Experiments (see Supplementary Information) to epimerize the C-16 stereochemistry using a number of bases and proton donors failed to produce any desired epimer 25a (Fig. 8 ). Next, intermediate 25 was converted to iodide 25b , aiming to alter the C-16 stereochemistry via radical reduction. Treatment of compound 25b with n -Bu 3 SnH failed again to provide 25a . Light-induced radical reductions were then attempted [97] . After extensive experiments (see Supplementary Information for details), we finally found that reduction of 25b with catalytic amount of [Ir(ppy) 2 (dtbbpy)]PF 6 in the presence of DIPEA and (TMS) 2 NH under blue LED (−60 °C) provided desired 25a in 47% yield (Fig. 8 ), with 25 being recovery in 16% yield. Deprotection of 25a with TFA followed by reduction with LiAlH 4 (LAH) gave natural koumidine 25c (80% yield over two steps) [98] , [99] . 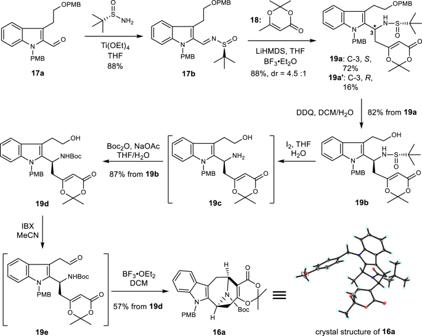Fig. 3: Gram-scale synthesis of common intermediate 16a. The key transformations to access the common intermediate16ainclude a vinylogous Mannich reaction of lithium dienolate18, and a Lewis acid mediated Mannich type cyclization of19e. Ac acetyl, Boct-butoxycarbonyl, DCM dichloromethane, DDQ 2,3-dichloro-5,6-dicyano-1,4-benzoquinone, IBXo-iodoxybenzoic acid, LiHMDS lithium bis(trimethylsilyl)amide, PMBp-methoxybenzyl, THF tetrahydrofuran. Fig. 8: Total synthesis of koumine-type alkaloids. Key transformations are light induced radical reduction of iodide 25b and NIS mediated cyclization of 37 to access koumine-type alkaloids. [Ir(ppy) 2 (dtbbpy)]PF 6 (4,4’-di- tert -butyl-2,2’-bipyridine)bis[(2-pyridinyl)phenyl]iridium(III) hexafluorophosphate, NIS N -iodosuccinimide, DIPEA N,N -Diisopropylethylamine. Full size image Treatment of the koumidine 25c with methyl chloroformate afforded amide 37 in 69% isolated yield. Reduction of 37 with LAH provided natural 19- Z -taberpsychine ( 13 , 78%) [100] . Although alkaloid koumine has been prepared by both partial synthesis and total synthesis in the literature [5] , [24] , [49] , [99] , cyclizations to construct the vicinal all-carbon quaternary centers in koumine-type structures generally followed the chemistry developed by Liu (SeO 2 /H 2 O, oxidation followed by cyclization in low yield) [101] and Sakai (Pd 0 , NaH in DMF, based on pre-synthesized 18-hydroxyl derivatives) [102] . Alternative way was reported recently via gold mediated indolyl addition to allene, and the cyclization adduct was converted to koumine in another five steps [49] . In this synthesis, we designed to fuse the two vicinal all-carbon quaternary centers via iodo-induced indolyl cyclization, as the resulting iodide ( 38 ) could be converted to olefin via elimination (Fig. 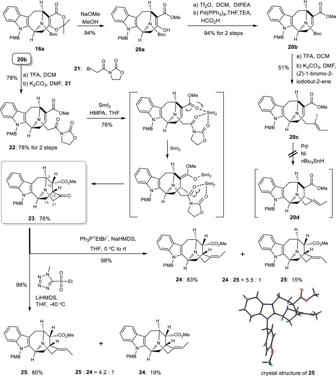Fig. 4: Synthesis of the common sarpagine type skeletons. After construction of the bridged E-ring via SmI2mediated SET reaction, the double bonds were assembled by Wittig reaction (E-selectivity) and Julia olefination (Z-selectivity). DIPEA diisopropylethylamine, DMFN,N-dimethylformamide, HMPA hexamethylphosphoramide, Me methyl, Ph phenyl, TEA triethylamine, Tf trifluoromethanesulfonyl, TFA trifluoroacetic acid, Et ethyl, NaHMDS sodium bis(trimethylsilyl)amide. 8 ). The amide 37 was thus treated with NIS in dichloromethane. To our delight, an efficient cyclization occurred, with iodide 38 being isolated as a single isomer in 88% yield. Treatment of iodide 38 with silver acetate in acetic acid furnished the olefin ( 39 ). After reduction of the amide bond with LAH, the first total synthesis of dihydrokoumine ( 40 ) was achieved. Oxidation of dihydrokoumine with PhIO in dichloromethane [49] afforded koumine in 98% yield. The NMR spectra of our synthetic alkaloids are consistent with those of the natural alkaloids [103] , [104] . We have developed a structure unit oriented strategy for the synthesis of cage-like Sarpagine-Ajmaline-Koumine type monoterpenoid indole alkaloids from readily available commercial materials. Among the natural alkaloids synthesized, eight molecules are synthesized for the first time. Key transformations developed are boron trifluoride etherate mediated tandem cascade cyclization to install the azabicyclo[3.3.1]nonane structure unit, samarium(II) iodide mediated SET cyclization to fuse the bridged-hexahydropyridine E-ring, trifluoromethanesulfonic acid induced cyclization to construct the all-carbon quaternary center in ajmaline-type alkaloids, and an efficient iodo-induced cyclization to establish the two vicinal all-carbon quaternary centers in the Koumine-type alkaloids. Our synthetic strategy provided a platform, enabling access to a wide variety of Sarpagine-Ajmaline-Koumine type natural products as well as their analogues, and should be found further application in the synthesis of bisindole alkaloids such as alstonisidine. General Melting points were measured on a Hanon MP 430 auto melting-point system and are uncorrected. The infrared (IR) spectra were recorded on a Nicolet iS10 FTIR spectrometer with 4 cm −1 resolution and 32 scans between wavenumber of 4000 cm −1 and 400 cm −1 . Samples were prepared as KBr disks with 1 mg of samples in 100 mg of KBr. 1 H-NMR and 13 C-NMR spectra were recorded on Bruker Avance 400 and 600 spectrometers. Chemical shifts are reported in parts per million (δ) referenced to tetramethylsilane (0.0 ppm), chloroform (7.26 ppm or 77.16 ppm), and methanol (3.31 ppm or 49.0 ppm), respectively. Data for 1 H-NMR and 13 C-NMR spectroscopy are reported as follows: chemical shift (δ ppm), multiplicity (s = singlet, d = doublet, t = triplet, q = quartet, m = multiplet, br = broad), coupling constant (Hz), integration. High Resolution Mass spectra were taken on AB QSTAR Pulsar mass spectrometer or Aglient LC/MSD TOF mass spectrometer. Optical rotations were recorded on a JASCO P-2000 polarimeter. All new compounds were characterized by IR, 1 H NMR, 13 C NMR, and HRMS. Silica gel (200–300 mesh) for column chromatography and silica GF 254 for TLC were obtained from Merck Chemicals Co. Ltd. (Shanghai). Anhydrous THF was dried by distillation over metallic sodium and benzophenone; dichloromethane, pyridine, and methanol were distilled from calcium hydride. Starting materials and reagents used in reactions were obtained commercially from Acros, Aldrich, and Adamas-beta ® , and were used without purification, unless otherwise indicated. 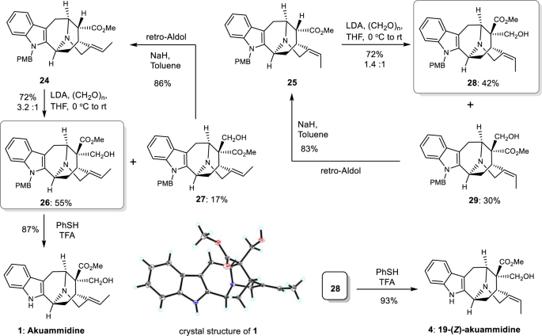Fig. 5: Synthesis of akuammidine (1) and 19-Z-akuammidine (4). Aldol condensation with formaldehyde. LDA lithium diisopropylamide. 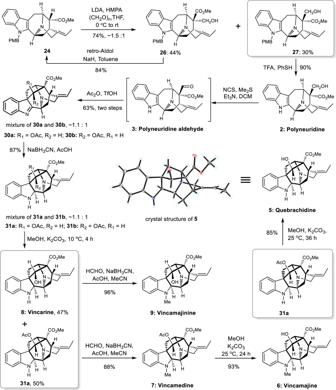Fig. 6: Synthesis of ajmaline type alkaloids. Quebrachidine, vincarine, vincamedine, and vincamajine were synthesized for the first time. NCSN-chlorosuccinimide. All reactions were conducted in dried glassware under a positive pressure of dry nitrogen or argon. Reagents and starting materials were accordingly transferred via syringe or cannula. 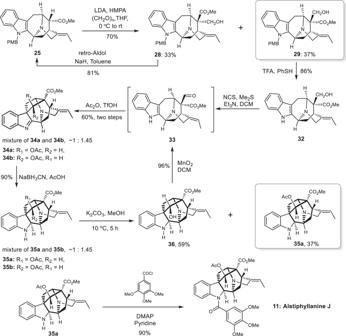Fig. 7: Synthesis of alstiphyllanine J. Alstiphyllanine J has a 19-Z-olefin moiety. DMAPN,N-4-dimethylaminopyridine. 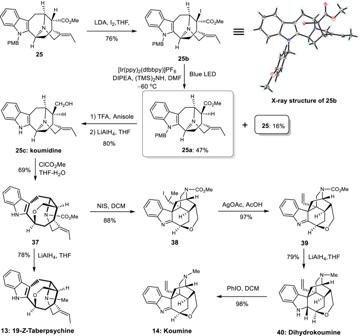Fig. 8: Total synthesis of koumine-type alkaloids. Key transformations are light induced radical reduction of iodide25band NIS mediated cyclization of37to access koumine-type alkaloids. [Ir(ppy)2(dtbbpy)]PF6(4,4’-di-tert-butyl-2,2’-bipyridine)bis[(2-pyridinyl)phenyl]iridium(III) hexafluorophosphate, NISN-iodosuccinimide, DIPEAN,N-Diisopropylethylamine. Reaction temperatures refer to the external oil bath temperature.